Evidence for methane production by saprotrophic fungi Methane in the biosphere is mainly produced by prokaryotic methanogenic archaea, biomass burning, coal and oil extraction, and to a lesser extent by eukaryotic plants. Here we demonstrate that saprotrophic fungi produce methane without the involvement of methanogenic archaea. Fluorescence in situ hybridization, confocal laser-scanning microscopy and quantitative real-time PCR confirm no contribution from microbial contamination or endosymbionts. Our results suggest a common methane formation pathway in fungal cells under aerobic conditions and thus identify fungi as another source of methane in the environment. Stable carbon isotope labelling experiments reveal methionine as a precursor of methane in fungi. These findings of an aerobic fungus-derived methane formation pathway open another avenue in methane research and will further assist with current efforts in the identification of the processes involved and their ecological implications. Methane (CH 4 ), the second most important anthropogenic greenhouse gas after CO 2 , is the most abundant reduced organic compound in the atmosphere and has a central role in atmospheric chemistry. The mixing ratio of CH 4 in the troposphere has increased from 715 p.p.b.v. in the preindustrial era to currently 1,800 p.p.b.v [1] , [2] . Global CH 4 emissions to the atmosphere amount to 500–600 Tg per year [3] . Large inter-annual variability in the annual growth rate of atmospheric CH 4 over the last 20 years [1] is a key issue in current research that remains unsolved [4] , [5] . A comprehensive understanding of the current global CH 4 budget including all its sources and sinks and the parameters that control its fluxes is a precondition to simulate past and future scenarios of its atmospheric mixing ratio. Traditionally, biogenic CH 4 was thought to be formed only by prokaryotic microorganisms (methanogens; archaea) under strictly anoxic conditions in wetland soils and rice paddies, the intestines of termites and ruminants, and human and agricultural waste [6] . However, recently CH 4 formation was also reported to occur under oxic conditions in terrestrial vegetation [7] , [8] and in animals [9] . The finding that dead and living plants can emit CH 4 under oxic conditions and without the intervention of microorganisms [7] , [8] , [10] justifies a search for other biotic but non-prokaryotic CH 4 sources in fungi and animals [11] . Less well known are the findings of Ghyczy et al . [9] , [12] who demonstrated that endothelial cells from rat liver produced CH 4 when exposed to site-specific inhibitors of the electron transport chain (ETC). A similar observation has been made for plant cell cultures grown under sterile and oxic conditions [13] . Hence, both plant and animal cells have been suggested to release CH 4 non-microbially. Fungi, another important kingdom of the eukaryotes, have not yet been investigated in terms of CH 4 formation. Fungi occupy a key role in degradation processes, representing an important part of the soil biome, and mycorrhizal fungi establish a close symbiosis with plant roots. Fungi have already been identified as members of a methanogenic food chain by providing methanogenic archaea with their substrate [14] , [15] , but they have to date not been reported to produce CH 4 per se. It is known that diverse bacteria can inhabit fungal mycelia [16] , [17] , [18] , but no methanogenic archaea have been found as endosymbionts in fungi. In this study, we investigated a broad range of saprotrophic fungi for their potential to produce CH 4 without participation of methanogens. To provide unambiguous evidence, we used the following criteria: observation of CH 4 production from eight Basidiomycetes grown under sterile conditions, verification that CH 4 is released from fungi employing isotopically labelled substrate, and confirmation of the absence of microbial contaminants using fluorescence in situ hybridization (FISH), confocal laser-scanning microscopy (CLSM) and quantitative real-time PCR. Furthermore, we discuss the relevance of our findings and their potential ecological implications for biogeochemical CH 4 cycling between ecosystems and the atmosphere. General results and information Several experiments with saprotrophic fungi grown on various substrates clearly demonstrated CH 4 production in the absence of methanogenic archaea ( Figs 1 , 2 , 3 ). The amount of CH 4 production varied between incubations ( Fig. 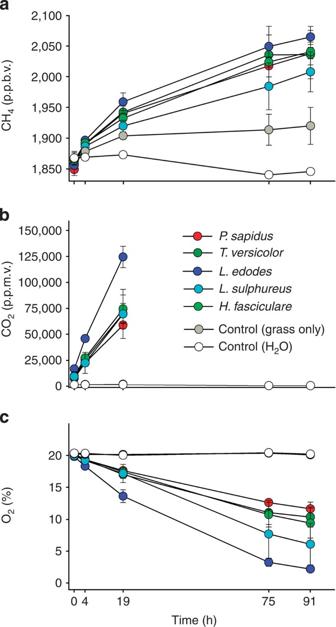Figure 1: Changes in headspace-gas mixing ratio. Mixing ratios of (a) CH4, (b) CO2and (c) O2in the flasks withP. sapidus, T. versicolor, L. edodes, L. sulphureusandH. fasciculare(n=3, controlsn=2) grown on grass. Error bars represent s.d. of mean for flasks containing fungi and range for controls. 1 ) and was related to CO 2 production ( Table 1 ), an indicator of metabolic activity and turnover. In general, initial atmospheric CH 4 mixing ratios at the start of incubations ranged from 1,800 to 2,000 p.p.b.v. The magnitude of CH 4 background levels complicated the detection of comparatively small increases of around 1 p.p.b.v. CH 4 per h. However, if the duration of the incubation was at least 24 h this was sufficient to detect CH 4 emissions, which were well above analytical thresholds. The increase in 13 CH 4 concentrations in samples where 13 C labelled glucose was used as a substrate indicated that the CH 4 formed was essentially the result of metabolism of substrate by fungi. All incubations were carried out under sterile and oxic conditions, that is, the O 2 mixing ratio in the flasks was always above 10% when CH 4 production occurred, except for the first experiment where fungi were cultured on grass ( Fig. 1 ). Here, in the flasks containing Laetiporus sulphureus and Lentinula edodes , O 2 mixing ratio dropped below 10% after 75 h incubation. Methane formation disappeared when fungi were heated at 100 °C in a water bath for several minutes (data not shown). Figure 1: Changes in headspace-gas mixing ratio. Mixing ratios of ( a ) CH 4 , ( b ) CO 2 and ( c ) O 2 in the flasks with P. sapidus, T. versicolor, L. edodes, L. sulphureus and H. fasciculare ( n =3, controls n =2) grown on grass. Error bars represent s.d. of mean for flasks containing fungi and range for controls. 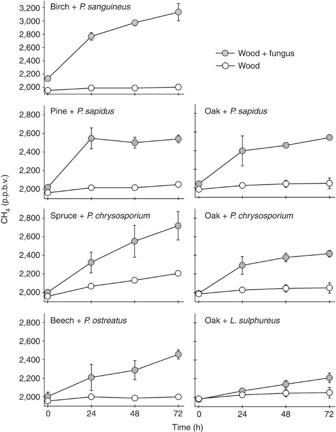Figure 2: CH4formation during wood decay. CH4-headspace mixing-ratio of wood-decaying fungi grown on different wood species (n=3except beech+P. ostreatuswheren=2). Error bars represent s.d. of mean for all examples except beech+P. ostreatuswhere error bars represent s.d. of the mean. Full size image Figure 2: CH 4 formation during wood decay. CH 4 -headspace mixing-ratio of wood-decaying fungi grown on different wood species ( n=3 except beech+ P. ostreatus where n=2 ). Error bars represent s.d. of mean for all examples except beech+ P. ostreatus where error bars represent s.d. of the mean. 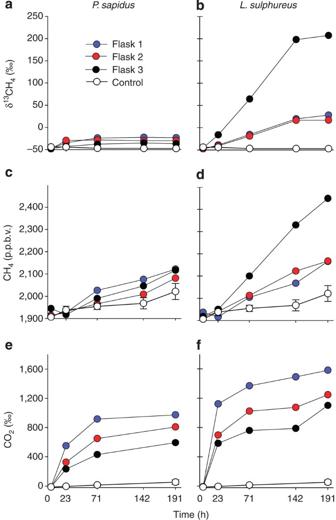Figure 3: Isotopic evidence for fungus-derived CH4formation. Stable carbon isotope values of CH4(a,b), CH4mixing ratios (c,d) and stable carbon isotope signature of CO2(e,f) in the headspace during the incubation ofL. sulphureusandP. sapiduson13C-labelled glucose. The control jars (n=3) contained sterile medium only. Error bars represent s.d. of mean. Full size image Figure 3: Isotopic evidence for fungus-derived CH 4 formation. Stable carbon isotope values of CH 4 ( a , b ), CH 4 mixing ratios ( c , d ) and stable carbon isotope signature of CO 2 ( e , f ) in the headspace during the incubation of L. sulphureus and P. sapidus on 13 C-labelled glucose. The control jars ( n =3) contained sterile medium only. Error bars represent s.d. of mean. Full size image Table 1 CH 4 :CO 2 -ratio of saprophytic fungi grown on different substrates ( n =3). Full size table CH 4 and CO 2 production by fungi When five saprotrophic fungi were grown separately on grass, a significant increase in the CH 4 mixing ratio occurred in all flasks ( Fig. 1a ). At the start of the incubation the mean CH 4 mixing ratio was approximately 1860 p.p.b.v. (atmospheric conditions). L. edodes showed the highest production rates (2.6±0.5 p.p.b.v. h −1 ), followed by Pleurotus sapidus (1.9±0.3 p.p.b.v. h −1 ), Trametes versicolor (1.7±0.5 p.p.b.v. h −1 ), Hypholoma fascicilore (1.2±0.3 p.p.b.v. h −1 ) and L. sulphureus (0.6±0.4 p.p.b.v. h −1 ). Differences between the five species were not significant. In the control 'grass' samples, CH 4 concentrations increased by an average rate of 1.6±0.2 p.p.b.v. h −1 ( r 2 =0.98), whereas in the control 'water only' the CH 4 mixing ratio slightly decreased over time. At the beginning of the experiment no significant differences in the initial CH 4 concentrations were detected due to the presence of the different fungi ( P= 0.294, one-way analysis of variance; ANOVA). However, after 4 h all fungi were significantly different from the controls, except for L. sulphureus (with the lowest production rates) that differed from the water control, but not from the grass control at 4 h and 19 h ( Fig. 1a ). The CO 2 mixing ratio ( Fig. 1b ) showed a rapid increase in the flasks with fungi, whereas no CO 2 increase occurred in the control samples of grass alone or water alone. As concentrations exceeded the measurement range after 19 h, the values were not recorded. The O 2 concentration steadily decreased over time in the flasks containing fungi, falling from 21% down to 3% in the case of L. edodes , whereas no change was noted in the controls ( Fig. 1c ). Methane formation of fungi grown on wood is presented in Fig. 2 and was in a range between 2.3 and 12.7 p.p.b.v. h −1 . From this figure it can be seen that the curve shapes would indicate saturation with time. For P. sapidus on pine the maximum CH 4 concentration is reached after 24 h incubation and therefore no CH 4 production rate is reported. Rates for the other fungi increased in the order: L. sulphureus on oak (2.3±0.6 p.p.b.v. h −1 ), Phanerochaete chrysosporium on oak (4.8±0.3 p.p.b.v. h −1 ), Pleurotus ostreatus on beech (5.5±1.4 p.p.b.v. h −1 ), P. sapidus on oak (5.6±0.3 p.p.b.v. h −1 ), P. chrysosporium on spruce (7.5±2.3 p.p.b.v. h −1 ) and Pycnoporus sanguineus on birch (12.7±1.5 p.p.b.v. h −1 ). Note that the CH 4 production rates are not related to fungal biomass. Significant CH 4 production was observed for 'spruce' wood without added fungi ( P= 0.004, tested via one-way ANOVA versus the control 'H 2 O only' (data not shown, no noteworthy changes in CH 4 concentration occurred)). Other wood species were not significantly different from the control 'H 2 O only', that is no CH 4 emissions occurred in the absence of fungi. Growth experiments using 13 C-labelled glucose Fungally derived CH 4 production on 13 C-labelled glucose substrate is presented in Fig. 3 . In all flasks containing fungi δ 13 C(CH 4 ) values increased with incubation time, whereas no 13 C enrichment occurred in the control flasks ( Fig. 3a,b ). For both species the increase of δ 13 C(CH 4 ) correlated with increasing CH 4 mixing ratios ( Fig. 3 and Supplementary Fig. S1 ). This correlation was strong for L. sulphureus ( r 2 =0.90; P <0.001, linear regression analysis) but due to the comparatively small increase in CH 4 amounts with P. sapidus cultures only a moderate correlation was noted ( r 2 =0.43, P =0.008, linear regression analysis). Considerable variation in the amount of CH 4 produced by the same species was observed. For example, an exceptionally high CH 4 formation was observed in one sample flask containing L. sulphureus , whereas CH 4 formation was two to three times lower in the other L. sulphureus sample flasks. Supplementation of fungi with 13 CH 3 -labelled methionine A likely precursor of CH 4 from fungi could be the thio-methyl group of methionine. Interestingly, this has recently been considered by Bruhn et al . [8] for the formation of CH 4 from living plants. To test this hypothesis for fungi ( P. sapidus) we employed methionine, which had only the carbon atom of the thio-methyl group (–S– 13 CH 3 ) labelled with 13 C. Immediately following addition of 13 C-methionine or unlabelled methionine the headspace gas of all samples showed δ 13 C(CH 4 ) values of around −46‰ (ranging from −45.4 to −47.1‰) and thus closely reflected the atmospheric background δ 13 C(CH 4 ) values of the laboratory air (−46.1±0.3). δ 13 C(CH 4 ) values for the headspace samples above fungi with added unlabelled methionine did not change significantly over the entire incubation period. In contrast, δ 13 C(CH 4 ) values in the headspace of P. sapidus supplemented with 13 C-methionine showed a continuous increase in δ 13 C(CH 4 ) values during the entire incubation period. A change in δ 13 C(CH 4 ) values of around 313 and 232‰ over the 30 h incubation period was measured ( Fig. 4 , n =2). On the basis of changes in CH 4 concentration and fungal dry weight measured after incubation, CH 4 formation was calculated to be 3.4±0.2 p.p.b.v. CH 4 h −1 g −1 . When the amount of 13 CH 4 was related to the total amount of CH 4 production 4.9 and 3.9% of headspace-CH 4 originated from the methyl group of methionine, respectively. These results suggest that the carbon atom of the sulphur-bound methyl group of methionine is a precursor of CH 4 generated by P. sapidus . 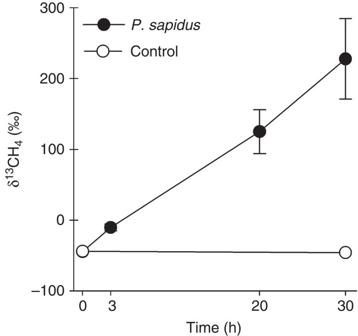Figure 4: Methionine as a precursor of CH4. δ13C signature of headspace-CH4whenP. sapiduswas grown on13C-methionine (n=2). Error bars represent s.d. of the mean. The control jars contained sterile medium only. Figure 4: Methionine as a precursor of CH 4 . δ 13 C signature of headspace-CH 4 when P. sapidus was grown on 13 C-methionine ( n=2 ). Error bars represent s.d. of the mean. The control jars contained sterile medium only. Full size image CH 4 to CO 2 ratio If CH 4 formation depends on metabolic activity it may in turn depend on factors such as fungal biomass, substrate availability, temperature and oxygen content. In the cultures with high CH 4 production more fungal biomass was visually observed. In addition, the CO 2 mixing ratio increases were smaller in cultures with a lower CH 4 production ( Fig. 1 ). The CH 4 /CO 2 ratios of six fungi grown on grass and/or 13 C-labelled glucose are presented in Table 1 . The CH 4 /CO 2 ratios ranged from 0.8 to 22.8×10 −6 . The CH 4 /CO 2 ratio for glucose was higher (that is, more CH 4 was produced per unit CO 2 ) than that for grass. Tests for microbial contamination Using FISH with probes for groups of archaea and bacteria, no such microorganisms could be detected in any of the tested cultures. Furthermore, several nucleic acid staining techniques were applied and analysed by epifluorescence microscopy. None of these methods revealed microbial contaminants in the culture medium, or microorganisms attached to the hyphae. For spatially resolved detection of potential non-fungal microorganisms, CLSM was employed. Imaging strategies comprised autofluorescence detection, a variety of nucleic acid stains and cell wall staining. Excitation with 405 nm did not show any autofluorescence signals in the region where the emission of methanogenic F 420 would be expected. Nevertheless, the fungal filaments showed some general cell internal autofluorescence. Nucleic acid staining was used as another test to search for possible microbial cells. Depending on the fluorochrome properties, the nucleic acid stains revealed internal features of fungal filaments ( Fig. 5 ). Some fluorochromes specifically stained the nucleus of fungi ( Fig. 5 ). However, none of the various fluorochromes indicated bacterial cells or even microcolonies. Cell wall staining proved the fungal filament structure and was employed in combination with nucleic acid stains ( Fig. 5 ). As a result, based on CLSM imaging, extracellular contamination of fungal cultures by archaea, bacteria or protists could be excluded. 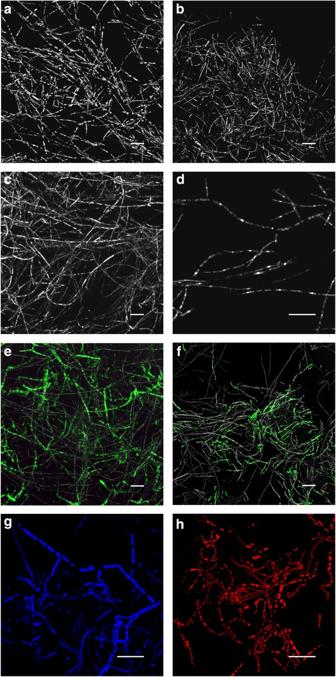Figure 5: Confocal laser-scanning microscopy. (a–d) Maximum intensity projection of fungal filaments fromL. sulphureus.Staining with different nucleic acid-specific fluorochromes is shown for Syto9 (a), SybrGreen (b), 4',6-diamidino-2-phenylindole (DAPI) (c) and Propidium iodide (d). To present the fluorescence emission signals with highest contrast, they are presented as measured by the photomultiplier in 8-bit grey scale. For clarity the reflection signal recorded for the samples inaandbwas removed. (e–h) Maximum intensity projection ofP. sapiduscultures including the reflection signal (e,f). Staining is shown for different nucleic acid-specific fluorochromes including Syto9 (e), SybrGreen (f), DAPI (g) and Propidium iodide (h). Colour allocation ineandf: Syto9/SybrGreen=green, reflection=grey; (g) DAPI=blue; (h) Propidium iodide=red. Please notice the heterogenic distribution of the nucleic acid signal, which is characteristic for many fungal strains. In addition, it is obvious that no bacterial signal is visible, neither as single cell, microcolony or associated with fungal filaments. Scale bars, 20 μm. Figure 5: Confocal laser-scanning microscopy. ( a – d ) Maximum intensity projection of fungal filaments from L. sulphureus. Staining with different nucleic acid-specific fluorochromes is shown for Syto9 ( a ), SybrGreen ( b ), 4',6-diamidino-2-phenylindole (DAPI) ( c ) and Propidium iodide ( d ). To present the fluorescence emission signals with highest contrast, they are presented as measured by the photomultiplier in 8-bit grey scale. For clarity the reflection signal recorded for the samples in a and b was removed. ( e – h ) Maximum intensity projection of P. sapidus cultures including the reflection signal ( e , f ). Staining is shown for different nucleic acid-specific fluorochromes including Syto9 ( e ), SybrGreen ( f ), DAPI ( g ) and Propidium iodide ( h ). Colour allocation in e and f : Syto9/SybrGreen=green, reflection=grey; ( g ) DAPI=blue; ( h ) Propidium iodide=red. Please notice the heterogenic distribution of the nucleic acid signal, which is characteristic for many fungal strains. In addition, it is obvious that no bacterial signal is visible, neither as single cell, microcolony or associated with fungal filaments. Scale bars, 20 μm. Full size image A quantitative real-time PCR with DNA from three flasks ( P. sapidus, P. chrysosporium, L. sulphureus ) was carried out to detect the McrA gene that encodes the methyl Coenzyme-M reductase. This enzyme is responsible for the last step in methanogenesis, the reduction of the Coenzyme-M bound methyl group to CH 4 . No evidence for such a product was detected in any of the fungal cultures, making contamination with methanogens implausible. A standard used as a positive control became amplified; therefore an error in PCR or PCR-solutions could be excluded. In addition, mycelia from the same cultures incubated in a medium for methanogens with acetate, methanol and H 2 /CO 2 as substrate under anaerobic conditions showed no turbidity or growth and the microscopic analysis (light and fluorescence microscopy [F 420 ]) was negative. Previous studies suggested that fungi enhance archaea-derived CH 4 formation by initiating the decay of organic matter, thereby providing methanogenic archaea with their substrate [15] , [19] . However, to our knowledge fungi have never been reported before as direct producers of CH 4 in the course of their own metabolism. In this study all fungi, that is eight saprotrophs, were found to produce significant amounts of CH 4 under oxic conditions. The magnitude of production was substrate-dependent, suggesting that this is likely a common process in all the fungal species employed in this study. Furthermore, CH 4 formation disappeared after inactivation of fungi at 100 °C for several minutes. These results suggest that intact fungal cells are involved in the formation of CH 4 . In a long-term experiment over several months during which fungi were grown on wood, CH 4 release was not associated with the generation or the existence of fungal fruiting bodies. Potential contamination of the fungal cultures with methanogens was carefully investigated. The results of CLSM ( Fig. 5 ), FISH, real-time PCR and cultivation attempts did not support any contention that the fungal cultures used for these investigations were contaminated with bacteria or methanogenic archaea, nor did they suggest the presence of methanogenic endosymbionts. In addition, the kinetics of CH 4 and CO 2 formations as well as O 2 decline did not indicate contamination with methanogenic archaea. When different fungi were grown on grass a correlation between CH 4 and CO 2 emissions and O 2 uptake was apparent ( Fig. 1 ). Fungal respiration processes require O 2 and deliver an equivalent amount of CO 2 . When the fungus was 'active', in terms of growth and metabolic processes, continuous release of CH 4 was observed. This relationship was best demonstrated by experiments with L. edodes, which showed the highest increase in CO 2 and CH 4 and the highest decrease in O 2 concentration. For each of the species after varying incubation periods the curve shapes for CH 4 release and O 2 consumption indicated saturation. This reflects a reduced decay of organic matter, most likely due to high CO 2 and low O 2 concentrations [19] . Owing to their natural habitat fungi have adapted their metabolic processes to suit reduced O 2 levels or high CO 2 mixing ratios, similar to those commonly found in laboratory incubation flask experiments, although differences between species do occur. For example, heart-rot fungi that grow at the centre of a tree trunk are more tolerant to low O 2 and high CO 2 conditions than the more surface-associated saprotrophic fungi [20] . However, in order to account for any possible negative effect of high CO 2 and low O 2 mixing-ratios on aerobic metabolic processes of the fungus during this study, concentrations >12% CO 2 and <9% O 2 were not considered when calculating production rates and hence the CH 4 /CO 2 ratios. Differences in the CH 4 /CO 2 ratios of fungi grown on grass or 13 C-labelled glucose ( Table 1 ) indicate a substrate-dependent release of CH 4 . However, the extent that the 'substrate' affects the CH 4 /CO 2 ratio and therefore CH 4 formation must be more carefully investigated with a broader range of substrates and this must await future studies. The CO 2 mixing ratio is also an indicator of microbial contamination in the control samples, as any microbial growth of heterotrophs would result in an immediate increase in the CO 2 mixing ratio. No such CO 2 increase was noted in any of the control samples ( Fig. 1 ). In the control 'grass' samples ( Fig. 1a ) the CH 4 mixing ratio increased without a concomitant increase in CO 2 . Thus, CH 4 released from the dead plant material resulted from the process shown by Keppler et al . [7] and Vigano et al . [21] Experiments in which labelled 13 C-glucose was supplied as a carbon source to the fungi not only unambiguously demonstrated that the CH 4 originated from the labelled substrate but also excluded any possibility of ingress from the laboratory atmosphere to the samples as the source of CH 4 . In addition, the laboratory atmosphere, which was measured alternately with every sample, never exceeded 2,000 p.p.b.v. CH 4 . The enrichment of 13 C in the produced CH 4 occurred simultaneously with the increase in the CH 4 mixing ratio ( Fig. 3 and Supplementary Fig. S1 ), indicating that fungal metabolism was directly involved in CH 4 formation. The biochemical pathway(s) involved in fungally derived CH 4 formation are currently unknown. Very recently it has been suggested [8] that the amino acid methionine might be a precursor for CH 4 formation in living plants. It is likely that methionine, a compound that also has a major role in sulphur metabolism and trans-methylation reactions in fungi, might act as a precursor compound of CH 4 formation. In this context, it can be readily envisaged that the thio-methyl group of methionine is a likely candidate carbon precursor of CH 4 formation in fungi. Experiments where 13 C-labelled methionine was added to P. sapidus showed that a fraction (~4–5%) of the produced methane must be derived from the supplemented thio-methyl group of methionine. Although there might be several mechanisms and other organic precursor compounds involved in aerobic CH 4 formation, these isotopic experiments convincingly indicate that the carbon atom of the sulphur-bound methyl group of methionine acts as a precursor of CH 4 in fungi. Our findings of an aerobic fungally derived CH 4 formation pathway may open another avenue in current CH 4 research concerning the processes involved and their ecological implications. So far, it is not clear if fungally derived CH 4 is a product of selection or a metabolic 'accident'. There is a possibility that CH 4 and CH 3 Cl production may be linked metabolically. The non-hymenochaetaceous white rot species P. chrysosporium and T. versicolor that were used in our studies are capable of biosynthesising CH 3 Cl as a biochemical methyl donor do not appear to release the compound during laboratory culture [22] . The observation should not be regarded as necessarily signifying that CH 3 Cl release from such species cannot occur in nature as the conditions and substrates normally employed for culture of these fungi in the laboratory bear little relation to those pertaining in their natural habitat [23] . However, growth of a hymenochaetaceous CH 3 Cl-releasing species such as Phellinus pomaceus on wood supplemented with sodium chloride yielded 8.5 μg h −1 over a 3-month period in laboratory studies [24] . This represents a CH 3 Cl production rate of approximately 1,000-fold higher than that observed for CH 4 release in this study. On cellulosic substrates supplemented with sodium chloride, rates of CH 3 Cl release by P. pomaceus were 4-fold higher than those with wood. Interestingly, the thio-methyl group of methionine has been shown to be a highly effective precursor of CH 3 Cl produced by the P. pomaceus . Thus, although there is a likely possibility that CH 4 formation could occur as a side reaction of CH 3 Cl biosynthesis in fungi, to fully explore this hypothesis would require a large set of experiments employing isotopically labelled compounds, including CH 3 Cl. Whiskerman et al . [13] who investigated sterile plant cell cultures suggested that CH 4 formation in living plants might be related to a site-specific disturbance of the ETC within the mitochondria. This is in accordance with the findings of Ghyczy et al . [9] , [12] who demonstrated that endothelial cells from rat liver produced CH 4 when exposed to site-specific inhibitors of the ETC. It would seem that aerobic CH 4 formation is not only a result of chemical formation from dead biomass as previously shown by several studies [8] , [11] but might also have a physiological role in eukaryotic groups such as fungi, animals and plants. For example aerobic CH 4 formation may be an integral part of cellular responses towards changes in oxidative status present in all eukaryotes. To test this hypothesis a broad range of biochemical experiments similar to those of Whiskerman et al . [13] need to be conducted. It is of interest to raise the question whether CH 4 formation by fungi may have an ecological function besides being a CH 4 source. It may act as a messenger molecule; however, this appears to be rather unlikely due to the high atmospheric mixing ratio of CH 4 . On the other hand, endogenous CH 4 production by fungi will likely affect methanotrophic communities. Our finding of a substrate-dependent release of CH 4 suggests a substrate-induced process involved in CH 4 formation. Possibly, N-availability or demand might affect CH 4 formation. There is evidence from the literature for an association of N 2 -fixing methylotrophic bacteria (that is, Methylocapsa acidophila and Methylocella palustris) in a wood block colonized by the Basidiomycete Hypholoma fasciculare [25] , [26] . Such an association may contribute to the ability of the fungus to produce CH 4 . Our results were obtained from a limited number of fungal cultures that were grown under sterile and controlled laboratory conditions. Therefore, an estimation of the magnitude of fungal-derived CH 4 formation and its significance for the global CH 4 budget would be speculative. At present, we do not know what physiological and environmental factors drive CH 4 emissions in nature. Thus, much more knowledge on effects of species and environmental controls are needed to estimate their true impact on the cycling of global CH 4 . Moreover, in nature it might be extremely difficult to distinguish between different CH 4 formation (and also consumption) processes as recently experienced with the formation of CH 4 from vegetation [8] , [11] . For example, Mukhin and Voronin [27] reported a wood decay-associated CH 4 formation caused by fungi in boreal forests. These authors suggested that fungi were not directly involved in the synthesis of CH 4 but they were necessary for its formation, by starting the food chain that leads to CH 4 -producing archaea [14] . Thus, they regarded it as a symbiotic association of wood-decaying fungi and anaerobic methanogenic microorganisms [28] but did not present any evidence for this mechanism. In our experiment where fungi were grown on diverse wood species ( Fig. 2 ), we provide evidence that aerobic CH 4 formation occurs during wood decay by saprophytic fungi without the help of archaea. Therefore, our results suggest that fungi were to some extent directly responsible for the observed CH 4 formation reported by Mukhin and Vronin [27] . However, our finding of CH 4 release by the control 'spruce' where no fungi were present highlights the difficulties to distinguish between different CH 4 sources in natural habitats. It is likely that a large part of fungally derived CH 4 is utilized by prevalent methanotrophs soon after its release, and thus gross CH 4 production by fungi will be difficult to measure in situ in ecosystems. Assessments of the CH 4 fluxes from an ecosystem shared by fungi and methanotrophs will only provide net CH 4 flux rates, which are the outcome of both processes, fungal (and in wet ecosystems of course archaeal) CH 4 production and simultaneous CH 4 consumption by methanotrophs [29] . It is conceivable that fungi enhance the CH 4 oxidation potential of an ecosystem by 'feeding' the methanotrophic community, thereby increasing their abundance. Evidence for a stimulation of CH 4 oxidation by endogenic CH 4 production via 'hot spots' (beetle larvae) was shown by Kammann et al . [30] for a grassland soil. The identification of fungal aerobic CH 4 formation may help to better understand global CH 4 oxidation patterns. Prince et al . [31] found highest net CH 4 consumption rates of up to 200 μg CH 4 m −2 h −1 in pristine forests, whereas anthropogenic land-use change degrades CH 4 oxidation [32] in the order pristine forests >managed forests >grasslands >crop fields (often near zero) [33] . This order corresponds to the amount of substrates that are likely available for saprotrophic fungi and hence endogenous CH 4 production to feed and sustain methanotrophic populations. The collective evidence from fungi, plants [7] and animal cells [9] indicates that aerobic CH 4 formation may not be an exotic process, but could be widespread in nature. Further research is needed to elucidate the mechanism of CH 4 formation in fungi and its possible relevance for ecology and the global CH 4 budget. Selected fungi In this study, eight Basidiomycetes from five different families were investigated for their capability to produce CH 4 . These were namely P. sapidus (Pleurotaceae, DSMZ 8266), L. sulphureus (Polyporaceae, DSMZ 1014), P. chrysosporium (Phanaerochaetaceae, FSU Jena L13-2), P. sanguineus (Polyporaceae, DSMZ 3023), P. ostreatus (Pleurotaceae, DSMZ 1020), T. versicolor (Polyporaceae, DSMZ 11269), H. fasciculare (Strophariaceae, DSMZ 2902) and L. edodes (Marasmiaceae, CBS 389.89). Fungi were chosen for their ecological and physiological characteristics or their well-established use in the laboratory (for example, uncomplicated cultivation, genome sequenced). According to Hintika [34] brown rot fungi grow even when the CO 2 concentration is as high as 70%. In contrast, the growth of litter decaying fungi is reduced at 20% CO 2 . L. sulphureus is also able to grow under very low oxygen conditions (that is O 2 <1%) [35] . Thus, this brown rot fungus is well adapted to low oxygen and high CO 2 concentration, that is, conditions that can occur in flasks during the incubations made during this investigation. Cultivation of fungi and incubation Wood, both dead and fresh green from different tree species, and grass from a garden lawn were used as substrate. Dead wood material (branches with 1.5–4 cm in diameter) was collected from the forest floor and shredded to small pieces (approx. 5 cm in length) with a shredder (Natura 1800L., Gloria, Witten, Germany), dried at 60 °C for 48 h and 100 g were stored in a flask (Weck, Hanau, Germany). The top 5 cm of a typical garden lawn (dominated by Lolium perenne ) was mechanically cut, homogeneously mixed and dried at 70 °C to constant weight. All substrates were either placed in 1 l, or, in the case of wood in 2.5 l, glass flasks (Weck, Hanau, Germany), closed with lids and rubber bands, and autoclaved. Each lid had a hole in the centre for gas exchange, which was sealed with a cotton stopper, or sealed air tight by fitting with a silicone stopper. Pure cultures of the fungi were added under sterile conditions. The sterile wood substrate was inoculated with a fungal submerged culture. Flasks containing agar medium were inoculated with small pieces of fungal pure cultures grown on agar plates. For trace gas measurements, the flasks were sealed with silicone stoppers equipped with a sampling port and Millex PTFE-sterile filters (0.22 μm, Millipore, Billerica, USA) to avoid contamination by indoor air during incubation and gas sampling. Subsequently, a gas sample was taken after flask closure. At each sampling point, volumes of either 20 ml (GC-analyses) or 60 ml [gas chromatography (GC) and isotope ratio mass spectrometry (IRMS) analyses] were removed from each flask and stored in air-tight 60 ml PE-syringes (Plastipak, BD, Franklin Lakes, USA) before analysis. For stable isotope measurements, 35 ml headspace gas samples were transferred into 12 ml Exetainers (Labco, High Wycombe, UK). Atmospheric air, the volume equivalent to that of the withdrawn sample, was added to each flask immediately after sampling. This dilution effect was taken into account when calculating mixing ratios and stable isotope values. All incubations were carried out at room temperature (21 °C). To account for the different amounts of fungal biomass in the flasks (which could not be analysed) and thus for potential differences in metabolic activity between species or replicates, CH 4 production was related to the CO 2 production by calculating the CH 4 /CO 2 ratios for each jar. The ratios enable differences caused by species or substrates to be evaluated. For this ratio only measurements at the beginning of the culture period, when the increase of CH 4 and CO 2 were linear, were considered. In all experiments where CH 4 production rates or the CH 4 /CO 2 ratio were used, only data sets where O 2 concentrations were above 10% are reported. For the calculation of fungal CH 4 production rates in the experiments 'grass' and 'wood' we accounted for possible CH 4 release by the growth substrates by subtracting the corresponding control from the samples containing fungi. Thus, the denoted rates reflect the difference between the control 'growth substrate' (here: wood or grass) and the fungus on respective growth substrate. To exclude CH 4 release from equipment, several rubber bands and silicone stoppers were placed in the 1 l flasks and incubated under identical conditions to those employed for the samples. Gas sampling after 5 days showed no increase in CH 4 concentration, that is artificial CH 4 release by the equipment could be excluded. Isotopic labelling of growth substrate The fungal growth medium consisted of yeast extract (2 g l −1 ), MgSO 4 (0.5 g l −1 ), KH 2 PO 4 (1.5 g l −1 ), variable C sources (20 g l −1 ) and micronutrients (ferric(III)chloride hexahydrate 0.08 g l −1 , zinc sulphate heptahydrate 0.09 g l −1 , manganese sulfate hydrate 0.03 g l −1 , copper sulfate pentahydrate 0.005 g l −1 , EDTA 0,4 g l −1 ), and was adjusted to pH 6.0. The glucose (Sigma-Aldrich, Steinheim, Germany) also contained 13 C glucose (isotec 99% 13C atoms, Sigma-Aldrich) in a ratio of 15:1, corresponding to a δ 13 C value of ~3,800‰. Each flask contained 0.5 mg of isotopically labelled glucose. Experiments using 13 C-labelled methionine A position-specific 13 C labelling experiment was conducted with methionine, which had only the carbon atom of the thio-methyl group (-S-methyl- 13 C) labelled with 13 C (99.9% enriched, Fa. Sigma). Methionine was added to the growth medium in a concentration of 0.125 g l −1 and P. sapidus was grown under sterile conditions for 4 days at 27 °C on a shaker before the incubation started. GC-analysis Gas samples were analysed within 36 h on a gas chromatograph (Shimadzu GC-14B, Kyoto, Japan) with a flame ionization detector (O 2 , CH 4 ) and an electron capture detector (N 2 O, CO 2 ) operated at 230 and 320 °C with N 2 as carrier gas (25 ml min −1 ) [30] , [36] . The length of the column (PorapakQ, Fa. Millipore, Schwallbach, mesh 80/100) was 3.2 m and 1/8 inch in diameter. The length of the precolumn was 0.8 m. The GC gas flow scheme and automated sampling was that of Mosier and Mack [37] and Loftfield et al . [38] , and peak area integration was undertaken with the Software PeakSimple, version 2.66. The s.d. of six atmospheric air standard samples was below 1.0%, 0.5%, 0.2% and 0.1% of their mean for CO 2 , N 2 O, CH 4 and O 2 , respectively. Stable carbon isotope analysis of CH 4 Gas samples with CH 4 mixing ratios of 1.8 to 2.5 p.p.m.v. were transferred to an evacuated 40-ml sample loop. Methane was trapped on Hayesep D, separated from interfering compounds by gas chromatography and transferred via an open split to the isotope ratio mass spectrometer (Thermo Finnigan Delta plus XL, Bremen, Gemany). All 13 C/ 12 C -isotope ratios are expressed in the conventional δ notation in per mil versus Vienna Peedee Belemnite (V-PDB), [‰] using the following equation: A tank of high-purity CO 2 (carbon dioxide 4.5, Messer Griesheim, Frankfurt, Germany) with a calibrated δ 13 C value of −23.63‰ (V-PDB) was used as a working reference gas (calibrated at MPI for Biogeochemistry in Jena, Germany). All δ 13 C values obtained from the analysis of CH 4 were corrected using three CH 4 working standards (Isometric instruments, Victoria, Canada) calibrated against International Atomic Energy Agency (IAEA) and National Institute of Standards and Technology (NIST) reference substances. The calibrated δ 13 C values of the three working standards in ‰ versus V-PDB were −23.9±0.2, −38.3±0.2 and −54.5±0.2‰. Statistics Treatment means and s.d. were calculated in Microsoft Excel 2007 (Redmond, USA) and error bars displayed in the figures are s.d.. One-way ANOVA (SigmaPlot 11.2.0.5, Systat Software Inc., San José, USA) was used to test for differences among fungal-, grass- and H 2 O-CH 4 -production separately for each treatment. For multiple comparisons of the fungus-inoculated jars versus the substrate-control jars 'grass' and 'H 2 O', the Holm–Sidak method was employed. The statistical evaluation of the 'wood decay' experiment and the 13 C-labelling experiments was carried out with SPSS Version 20.0. To test for differences between the controls 'wood' and the 'H 2 O' (data not shown) one-way ANOVA with Dunnett-T3 as a Post-Hoc test was used. The correlation between 13 C signature increase and CH 4 concentration increase were tested via linear regression analysis. Differences at the P <0.05 level were reported as significant. Tests for microbial contamination A detailed description of FISH, CLSM, PCR diagnostics and cultivation approaches of archaea is given in the supplementary information online. How to cite this article: Lenhart, K. et al . Evidence for methane production by saprotrophic fungi. Nat. Commun. 3:1046 doi: 10.1038/ncomms2049 (2012).